Discovery of a novel methanogen prevalent in thawing permafrost Thawing permafrost promotes microbial degradation of cryo-sequestered and new carbon leading to the biogenic production of methane, creating a positive feedback to climate change. Here we determine microbial community composition along a permafrost thaw gradient in northern Sweden. Partially thawed sites were frequently dominated by a single archaeal phylotype, Candidatus ‘ Methanoflorens stordalenmirensis ’ gen. nov. sp. nov., belonging to the uncultivated lineage ‘Rice Cluster II’ (Candidatus ‘ Methanoflorentaceae ’ fam. nov.). Metagenomic sequencing led to the recovery of its near-complete genome, revealing the genes necessary for hydrogenotrophic methanogenesis. These genes are highly expressed and methane carbon isotope data are consistent with hydrogenotrophic production of methane in the partially thawed site. In addition to permafrost wetlands, ‘ Methanoflorentaceae ’ are widespread in high methane-flux habitats suggesting that this lineage is both prevalent and a major contributor to global methane production. In thawing permafrost, Candidatus ‘ M. stordalenmirensis ’ appears to be a key mediator of methane-based positive feedback to climate warming. High northern latitudes are disproportionately affected by global climate change with the effects of warming already evident in the decline of permafrost [1] , [2] . Rising temperatures can initiate ecosystem transition from intact permafrost to wetland, with a concomitant increase in the emission of the potent greenhouse gas methane [2] , [3] , [4] . Microbial populations are thought to be primarily responsible for methane production in thawing permafrost, yet remain largely unstudied [5] . The Stordalen Mire environment in northern Sweden represents a thaw gradient, with its ecosystem divided into three habitat stages: palsa (intact permafrost), bog (partially thawed) and fen (fully thawed) [3] , [6] , [7] , facilitating its use as a model ecosystem for studying methane generation associated with thawing peat. From 1970 to 2000, the intact palsa receded 10% while the bog and fen areas expanded 12% (refs 6 , 7 ) resulting in the mire’s net methane emission increasing by up to 66% (refs 3 , 7 ). Microbial populations that drive methane production in thawing permafrost influence the magnitude and trajectory of methane-based climate feedbacks [5] . Here we show that microbial communities in the active layer of thawing and thawed Stordalen Mire sites are often dominated by a single archaeal phylotype. Culture-independent recovery of the near-complete genome of this archaeon revealed the metabolic potential for hydrogenotrophic methanogenesis. Pore water methane concentrations and isotopic composition, coupled with metaproteomic analyses confirm the methanogenic activity of this organism primarily via the hydrogenotrophic pathway. Furthermore, members of this methanogenic lineage are prevalent and widely distributed across arctic ecosystems and are likely major contributors to global methane generation. Thawing mire permafrost is dominated by a single methanogen Stordalen Mire is instrumented to measure methane fluxes from the three thaw-sequence habitats via an autochamber system [8] . As observed previously, methane flux was emitted from the waterlogged bog and fen sites, with none detectable from the drier palsa ( Fig. 1c ). Microbial communities surrounding each habitat’s autochambers, and in several matched sites nearby, were sampled at three depths in triplicate in 2010 ( Supplementary Data 1 ), during the typical seasonal methane emission maximum, and over the 2011 seasonal thaw (June to October). 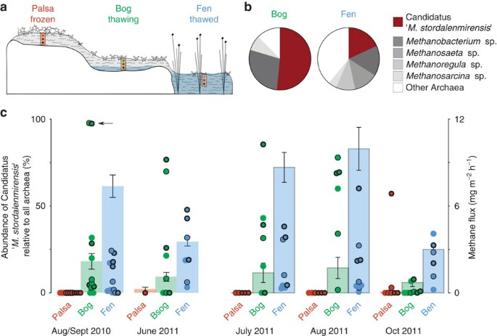Figure 1: Seasonal abundance ofCandidatus‘M. stordalenmirensis’ along a thaw gradient. (a) Schematic of the sampling sites at Stordalen Mire, Sweden; the white area indicates permafrost, hashed area indicates the active layer and blue area indicates water. Boxes denote coring sites and coloured dots represent the sampling site and depth: intact (brown), thawing (green) and thawed (blue), and thick, thin and no borders representing deep, middle and surface, respectively. (b) Relative abundance of dominant methanogens in the bog and fen sites, compared with the total number of archaeal sequences. (c) Relative abundance of ‘M. stordalenmirensis’ in microbial communities between 2010 and 2011. Coloured dots represent sampling site and depth: intact (brown), thawing (green) and thawed (blue), and thick, thin and no borders representing deep, middle and surface, respectively. Arrow indicates the two samples used for metagenomic sequencing. Histograms indicate associated methane flux for each site averaged across the week before cores were taken (2010 and June 2011 represent a 10 year flux average7, July–October 2011 measuredin situ). All error bars represent s.e. Communities were initially profiled using culture-independent small subunit (SSU) rRNA amplicon pyrosequencing ( Supplementary Table 1 ; Supplementary Data 1 ). Archaeal populations in the thawing and thawed sites were frequently dominated by a single archaeal phylotype, on average comprising 27% and up to 98% of archaeal reads ( Fig. 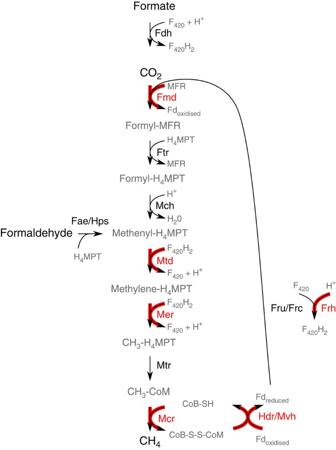Figure 2: Hydrogenotrophic methanogenesis pathway encoded inCandidatus‘M. stordalenmirensis’. The complete pathway is typical of methanogens lacking cytochromes with the exception of a missing Eha/Ech hydrogenase, which may be substituted with a novel hydrogenase. Highly expressed proteins detected in the metaproteomic data are indicated in red. 1 ; Supplementary Table 2 ). This archaeal phylotype was primarily observed in deeper more anoxic samples and was almost entirely absent from oxic zones ( Fig. 1 ), suggesting that it may be influenced by oxygen concentration. There appears to be a seasonal effect with higher relative abundance during June to August 2011, the warmest months of summer, and lower abundance in October suggesting that temperature may also be an important determinant of population dynamics. Figure 1: Seasonal abundance of Candidatus ‘ M. stordalenmirensis ’ along a thaw gradient. ( a ) Schematic of the sampling sites at Stordalen Mire, Sweden; the white area indicates permafrost, hashed area indicates the active layer and blue area indicates water. Boxes denote coring sites and coloured dots represent the sampling site and depth: intact (brown), thawing (green) and thawed (blue), and thick, thin and no borders representing deep, middle and surface, respectively. ( b ) Relative abundance of dominant methanogens in the bog and fen sites, compared with the total number of archaeal sequences. ( c ) Relative abundance of ‘ M. stordalenmirensis ’ in microbial communities between 2010 and 2011. Coloured dots represent sampling site and depth: intact (brown), thawing (green) and thawed (blue), and thick, thin and no borders representing deep, middle and surface, respectively. Arrow indicates the two samples used for metagenomic sequencing. Histograms indicate associated methane flux for each site averaged across the week before cores were taken (2010 and June 2011 represent a 10 year flux average [7] , July–October 2011 measured in situ ). All error bars represent s.e. Full size image Comparative sequence analysis placed the dominant archaeal phylotype in a euryarchaeal clade with no cultivated representatives, Rice Cluster II (RC-II) [9] , [10] , within the class Methanomicrobia . Given the dominance of this population and its phylogenetic association with known methanogens ( Supplementary Fig. 1 ), we sought to gain initial insight into its metabolic potential by recovering its genome through shotgun metagenomic sequencing. Over 500 Mbp of Ion Torrent PGM sequence data (single-end 100 bp reads) were obtained from the two bog samples most enriched in RC-II ( Fig. 1 ), and almost all of the archaeal SSU rRNA reads extracted from the metagenome belonged to this clade. Assembly and binning (see Methods) recovered the RC-II population genome in 117 contigs. Ion Torrent mate-pair sequencing (452 Mbp, insert size 2–3 kbp) linked these contigs into 10 scaffolds with a combined length of 2.1 Mbp and an average G+C content of 52%. This draft genome is near-complete and derived from a single population based on recovery of a complete set of 104 conserved archaeal marker genes [11] identified in single copy. This is the first reported genome recovered from metagenomic data generated exclusively on the Ion Torrent PGM platform. A genome tree constructed from conserved marker genes ( Supplementary Fig. 1 ) indicates that the organism is a member of the order Methanocellales [12] refining its placement based only on the SSU rRNA gene [13] . Given its phylogenetic position and high abundance in thawing permafrost, we propose the name Candidatus ‘ Methanoflorens stordalenmirensis ’ gen. nov., sp. nov. as the first representative of a new family, Candidatus ‘ Methanoflorentaceae ’ fam. nov. Candidatus ‘ M. stordalenmirensis ’ is an active methanogen Metabolic reconstruction of the Candidatus ‘ M. stordalenmirensis ’ genome revealed all of the genes required for hydrogenotrophic methanogenesis from carbon dioxide, formate and formaldehyde ( Fig. 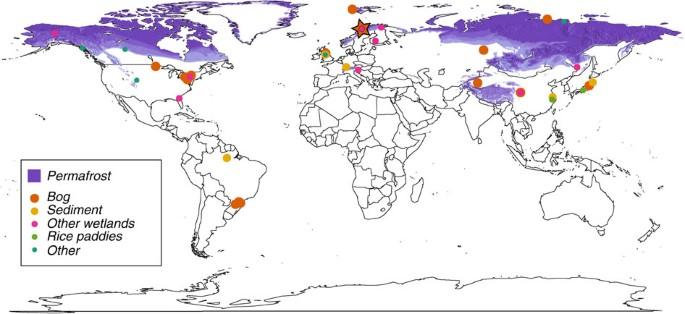Figure 3: Global distribution ofCandidatus‘M. stordalenmirensis’-like sequences. Each dot represents an instance where one or more publishedSSU rRNAgene sequences with >97% identity to ‘M. stordalenmirensis’ was observed. Dots are colour coded according to ecosystem type, and the star indicates Stordalen Mire. Purple shading indicates permafrost distribution and classification. This figure was drawn using the R58package ‘maps’ version 2.2-6 (http://cran.r-project.org/web/packages/maps/) then modified with Gimp (gimp.org) and Inkscape (inkscape.org). Overlayed permafrost distribution was derived fromhttp://svs.gsfc.nasa.gov/goto?3511(NASA/Goddard Space Flight Center Scientific Visualization Studio, National Snow and Ice Data Center, World Data Center for Glaciology). 2 ; Supplementary Table 3 ). This is consistent with pore water isotopic ratios (δ 13 C CH4 =−79 to −90), which indicate that most of the methane (~130–170 mM) is produced via hydrogenotrophic methanogenesis in bog sites, where Candidatus ‘ M. stordalenmirensis ’ is in high abundance relative to other methanogens ( Supplementary Tables 4 and 5 ). One difference between the canonical hydrogenotrophic methanogenesis pathway and that reconstructed from the Candidatus ‘ M. stordalenmirensis ’ genome is the lack of discernable Ech or Eha hydrogenases that provide sub-stoichiometric amounts of the reduced ferredoxin necessary for the reduction of carbon dioxide ( Fig. 2 ) [14] , [15] . A distantly related putative hydrogenase with no known archaeal orthologues was identified, which may fulfil this function ( Supplementary Table 3 ), although we cannot rule out that Eha or Ech hydrogenases may be encoded in the small unassembled portions of the genome. Methanogens can also be distinguished based on whether they use cytochromes. In contrast to previous reports that methanogens with cytochromes predominate in cold environments [14] , no cytochromes were identified in the Candidatus ‘ M. stordalenmirensis ’ genome including the cytochrome-containing hydrogenase complex ( vhtACG / hdrDE ), which is present in other members of the order Methanocellales and the sister order Methanosarcinales ( Supplementary Fig. 1 ). Figure 2: Hydrogenotrophic methanogenesis pathway encoded in Candidatus ‘ M. stordalenmirensis ’. The complete pathway is typical of methanogens lacking cytochromes with the exception of a missing Eha/Ech hydrogenase, which may be substituted with a novel hydrogenase. Highly expressed proteins detected in the metaproteomic data are indicated in red. Full size image To assess the in situ activity of Candidatus ‘ M. stordalenmirensis ’, we determined the metaproteome and pore water methane concentration of a fen sample from 2010. Candidatus ‘ M. stordalenmirensis ’ comprised 7.6% of the community proteome based on relative abundance from spectral counts ( Supplementary Table 6 ), likely reflecting its lower relative abundance at this site (8%; Supplementary Data 1 ). Of the identified Candidatus ‘ M. stordalenmirensis ’ proteins, ~64% were involved in hydrogenotrophic methanogenesis (red proteins in Fig. 2 ; determined based on spectral counts). Pore water measurements confirmed that the fen sample was methane rich (201±48 μM) ( Supplementary Table 5 ). The metabolic reconstruction, along with methane concentrations, isotopes and proteomic data, taken together with its distribution along the thaw gradient ( Fig. 1 ) indicate that Candidatus ‘ M. stordalenmirensis ’ is a major contributor to total methane production in Stordalen Mire. Methanoflorentaceae are globally distributed Mackelprang et al. [16] reported the draft archaeal genome of a novel methanogen enriched in Alaskan permafrost soil from Hess Creek thawed artificially over 7 days. Several of the contigs from this draft genome were most similar to Candidatus ‘ M. stordalenmirensis ’ (average nucleotide identity of best hits 79%). A partial methyl-coenzyme A reductase ( McrA ) gene identified on one of these contigs has 99% amino-acid sequence similarity to its homologue in Candidatus ‘ M. stordalenmirensis ’. However, we were unable to confirm the specific relationship between the two populations as no SSU rRNA gene was found in the Hess Creek genome, and of the 104 single-copy genes used for genome validation, 50 exist in more than one copy in the Hess Creek archaeon ( Supplementary Table 7 ), indicating a probable co-assembly of multiple populations. Despite these complications, the inferred presence of a member of the ‘ Methanoflorentaceae’ in Hess Creek, a geochemically distinct and geographically remote environment to Stordalen Mire, suggest that this lineage may be a key contributor to methane flux in thawing permafrost worldwide. Candidatus ‘ M. stordalenmirensis ’-like organisms have been observed in other Arctic wetlands and across the geographic range of wetland ecosystems. Sequences with ≥97% identity to the Candidatus ‘ M. stordalenmirensis ’ SSU rRNA gene are present in the non-redundant nucleotide database from 33 locations across four continents ( Fig. 3 ) comprising up to 75% of detected archaeal sequences in some instances [17] . These locations include temperate, subtropical and marine habitats spanning a wide range of physicochemical conditions ( Supplementary Tables 8 and 9 ). The pH of these locations range from ~4 to 7, similar to the pH range of the Stordalen Mire samples where Candidatus ‘ M. stordalenmirensis ’ was observed ( Supplementary Table 10 ). A unifying feature of these habitats is demonstrable or putative methane flux; most were wetlands associated with Sphagnum or graminoid vegetation. This provides further evidence that ‘ Methanoflorentaceae ’ likely are important contributors to global methane generation. Figure 3: Global distribution of Candidatus ‘ M. stordalenmirensis ’-like sequences. Each dot represents an instance where one or more published SSU rRNA gene sequences with >97% identity to ‘ M. stordalenmirensis ’ was observed. Dots are colour coded according to ecosystem type, and the star indicates Stordalen Mire. Purple shading indicates permafrost distribution and classification. This figure was drawn using the R [58] package ‘maps’ version 2.2-6 ( http://cran.r-project.org/web/packages/maps/ ) then modified with Gimp (gimp.org) and Inkscape (inkscape.org). Overlayed permafrost distribution was derived from http://svs.gsfc.nasa.gov/goto?3511 (NASA/Goddard Space Flight Center Scientific Visualization Studio, National Snow and Ice Data Center, World Data Center for Glaciology). Full size image Microorganisms play a central role in the carbon cycle and therefore it is important to understand their contribution to climate change feedback. However, our knowledge of the microbiology underpinning carbon cycling, in particular methane production and consumption, is still developing [5] , [18] , [19] , [20] . Permafrost constitutes a large reservoir of cryo-sequestered carbon that is currently being made bioavailable by climate change-induced thaw and subsequently released into the atmosphere through biogenic conversion to carbon dioxide and methane [21] , [22] , [23] . The chronosequence present at Stordalen Mire in northern Sweden is a model system for studying permafrost thaw. Here, we characterized the microbial community along the thaw gradient, finding that a novel archaeal phylotype is present at high abundance and is likely responsible for a significant proportion of the increasing amounts of methane being released from the mire. We obtained a high-quality draft population genome of a representative of this lineage, Candidatus ‘ M stordalenmirensis ’, and confirmed its ability to produce methane hydrogenotrophically in thawing permafrost at the mire. If the contribution of Candidatus ‘ M. stordalenmirensis ’ to ecosystem methane emissions is proportional to its relative abundance, as suggested by metaproteomic and isotope data, then it is responsible for producing a sizable amount of methane at the mire and is a major contributor to warming. The discovery of a globally distributed methanogenic lineage, the ‘ Methanoflorentaceae ’, that seasonally blooms in response to permafrost thaw suggests that these archaea are substantial contributors to positive feedback in climate change. Methanogenesis is the final step in the degradation of both cryo-sequestered and recently fixed carbon, however, the community members that provide the necessary precursors for methanogenesis in thawing permafrost are currently unknown [24] , [25] , [26] . Similarly, methanotrophs may play a substantial role in limiting methane emission from thawing permafrost and their distribution and activity also warrants investigation, for example refs 27–29. Such contextualized understanding of the ‘ Methanoflorentaceae ’ should improve model predictions for future feedbacks to climate change. Sampling Sampling dates and locations are detailed in Supplementary Table 10 . Triplicate soil cores were collected using a push corer from palsa (intact permafrost), bog (partially thawed) and sedge-dominated ( Eriophorum spp.) fen in Stordalen Mire, northern Sweden (68°21′N, 19°03′E, 359 m a.s.l.) on 30th September and 1st August 2010, and 15th June, 12th July, 16th August and 16th October 2011. Cores were subsampled by depth (see Supplementary Table 10 ), avoiding 1 cm around the edge of the corer, placed in cryotubes, saturated with ~3 volumes LifeGuard solution (MoBio Laboratories, Carlsbad, CA, USA) and stored at −80 °C until processing. Pore water measurements Pore water samples were collected from 35 to 40 cm below the peat surface using a syringe connected to a stainless steel tube. Samples were filtered with 25-mm diameter Whatman Grade GF/D glass microfiber filters (2-μm particle retention) and injected into 30 ml evacuated vials sealed with butyl rubber septas. Samples were frozen and shipped to Florida State University for analysis. After thawing, samples were acidified with 0.5 ml of 21% H 3 PO 4 and the headspace was brought to atmospheric pressure with helium. The sample headspace was analysed for concentrations, δ 13 C of CH 4 and CO 2 on a continuous-flow Hewlett-Packard 5890 gas chromatograph (Agilent Technologies) at 40 °C coupled to a Finnigan MAT Delta V isotope ratio mass spectrometer via a Conflo 2 interface system (Thermo Scientific, Bremen, Germany). The headspace gas concentrations were converted to pore water concentrations based on their known extraction efficiencies, defined as the proportion of formerly dissolved gas in the headspace. An extraction efficiency of 0.95 (based on repeated extractions) was used for CH 4 , and the extraction efficiency for CO 2 relative to DIC was determined based on CO 2 extraction from dissolved bicarbonate standards [30] . The carbon isotope fractionation factor ( α c ) was calculated as in Whiticar et al. [31] : The standard errors for α C were propagated from the δ 13 C errors as follows: where , and are the s.e. for α c , δ 13 C DIC and δ 13 C CH 4 , respectively. pH of the pore water was collected in the field with a Cole-Parmer portable pH meter. Methane flux measurements The autochamber system at Stordalen Mire has previously been described in detail [8] . Briefly, a system of eight automatic gas-sampling chambers made of transparent Lexan was installed in the three habitat types at Stordalen Mire in 2001 ( n =3 each in the palsa and bog habitats, and n =2 in the fen habitat). Chambers cover an area of 0.14 m 2 (38 cm × 38 cm), with a height of 25–45 cm. Each chamber is closed once every 3 h for a period of 5 min. The chambers are connected to the gas analysis system, located in an adjacent temperature controlled cabin, by 3/8 inch Dekoron tubing through which air is circulated at ~2.5 l min −1 . During the 2011 season, the system was updated with a new chamber design similar to that described by Bubier et al. [32] The new chambers cover an area of 0.2 m 2 (45 cm × 45 cm), with a height ranging from 15 to 75 cm depending on habitat vegetation. At the palsa and bog sites, the chamber base is flush with the ground and the chamber lid (15 cm in height) lifts clear of the base between closures. At the fen site, the chamber base is raised 50–60 cm on lexon skirts to accommodate large stature vegetation. Starting July 1st 2011, methane fluxes were measured using a Quantum Cascade Laser Spectrometer (QCLS, Aerodyne Research Inc.). The QCLS instrument deployed at Stordalen Mire is a modification of the technology described in detail by Santoni et al. [33] We connected the QCLS to the main autochamber circulation using ¼ inch Dekoron tubing and a solenoid manifold that enables selection between the autochamber flow and an array of calibration tanks. During measurement periods, filtered (0.45 μm, teflon filter) and dried (Perma Pure PD-100 T-24MSA) sample-air flows at 1.4 SLPM through the 2-l QCLS sample cell volume at 5.6 kPa. A downstream solenoid controls the QCLS return flow so that air only recirculates during autochamber measurement periods; during calibration periods tank air is vented to the room. Calibrations were done every 60 min using three calibration gases spanning the observed concentration range (1.5–10 p.p.m.). For each calibration period a linear calibration curve was fitted and the fit parameters were linearly interpolated between calibration periods. For each autochamber closure fluxes were calculated using a method consistent with that detailed by Bäckstrand et al. [8] using a linear regression of changing headspace CH 4 concentration over a period of 2.5 min. Eight 2.5-min regressions were calculated, staggered by 15 s and the most linear fit (highest r 2 ) was then used to calculate flux. Average fluxes were calculated for the week leading up to and including the sample collection dates based on indivdual chambers as the unit of replication ( n =3 for palsa and bog, n =2 for fen). For sampling dates before the installation of the QCLS, CH 4 fluxes were estimated from the CH 4 flux data published by Bäckstrand et al. [7] Characteristic fluxes for the week leading up to and including the August/September 2010 sampling (day of year 238–244) and June 2011 sampling (day of year 160–166) were calculated by averaging flux measurements for those dates from the 2002 to 2007 data set using individual chambers as the unit of replication. SSU rRNA gene amplicon sequencing Total nucleic acids were extracted from ~2 g peat sample using the PowerMax Total Nucleic Acid extraction kit (MoBio), retaining the LifeGuard preservation solution during lysis. DNA was purified by RNaseA digestion, phenol-chloroform-isoamyl alcohol purified and ethanol precipitated. Approximately 15 ng DNA from each sample was used as a template in PCR reactions. The universal primers, 926F (5′- CCTATCCCCTGTGTGCCTTGGCAGTC TCAG AAACTYAAAKGAATTGRCGG-3′, sequencing adapter in bold, key underlined and SSU-specific primer following) and 1392wR (5′- CCATCTCATCCCTGCGTGTCTCCGAC TCAG XXXXXACGGGCGGTGWGTRC-3′, as above but also included a variable length multiplex identifier unique to each sample (Xs) listed in Supplementary Table 11 ), were used to amplify an ~500 bp (V6–V8) region of the SSU rRNA gene from community members (similar to a primer set tested in Engelbrektson et al. [34] ). These primers were confirmed to match exemplar strains from each of the currently known [35] seven orders of methanogens (IMG 4.1 (ref. 36) [36] identifier 2518645582, IMG 4.0 identifiers 637000162, 649633067, 2512564055, 638154507, 640753014 and 638154506) using iPCRess 2.2.0 (ref. 37) [37] . Template DNA was amplified in duplicate 50 μl reactions containing 1 U Taq DNA polymerase (Fisher), 0.2 mM dNTP mix (Fisher), 2 mM MgCl 2 (Fisher), 2 μM of each primer and 10 μg μl −1 BSA (NEB). PCR was in a Veriti thermocycler (AppliedBiosystems, Carlsbad, CA, USA) with an initial denaturation step of 95 °C for 3 min, 30 cycles of dissociation at 95 °C for 30 s, annealing at 55 °C for 45 s, extension at 74 °C for 30 s and final extension of 10 min at 74 °C. Amplicons were sequenced using the reverse primer on the 454 GS FLX (Roche) with samples unrelated to this study using equal volumes. Informatic analysis methods are detailed in Supplementary Methods . Samples were multiplexed over five separate runs. Metagenome sequencing For metagenomic sequencing, ~100 ng DNA was sheared using a Covaris S2 (Covaris Inc.) according to the methods outlined in the Ion Fragment Library Kit protocol (publication 4467320 Rev. B). The library was prepared using the Ion Plus Fragment Library Kit and a modified version of the method described in the corresponding user guide (publication 4471989 Rev. B). After the size and concentration of the libraries was determined using the Agilent 2100 Bioanalyzer (Agilent Technologies) with the High Sensitivity DNA Kit (Agilent Technologies), the library was diluted and the Ion OneTouch system was used to prepare the template, using the Ion OneTouch Template Kit and corresponding user guide (publication 4468007 Rev. E). Sequencing of three 316 chips was performed using the Ion Sequencing Kit and associated user guide (publication 4469714 Rev. C). The Ion Torrent Suite version 2.0 and 2.0.1 were used for analyses and the SFF was subsequently downloaded for analysis. Genome assembly and binning A total of 533 Mb of single-ended 100 bp Ion Torrent PGM shotgun data were generated. Fastq and XML files were extracted from the SFF using sff_extract ( http://bioinf.comav.upv.es/sff_extract ) version 0.2.12 using parameters ‘-Q -s metagenome2.fastq -x metagenome2.xml 1.sff 2.sff 3.sff’. To determine SSU rRNA sequences detected from this set, reads were mapped using BWA-MEM (v0.7.5a) against the GreenGenes 2013 (ref. 38) [38] database 97% representative set. 98% of primary Archaeal hits that were >95% identical over at least 95 bp were assigned to Candidatus ‘ M. stordalenmirensis ’. Extracted sequences were assembled using MIRA [39] 3.4.0 with parameters ‘--project=metagenome2 --job= denovo ,genome,accurate,iontor -MI:sonfs=no’. Contigs with coverage between 22 and 36 were considered for further analysis based on the method by Teeling et al. [40] and implemented here as a biogem [41] called bio-kmer_counter ( https://github.com/wwood/bioruby-kmer_counter ) and visualized using ggplot2 (ref. 42 ) ( Supplementary Fig. 2 ). Reads included in the assembly in the remaining 154 contigs were extracted and re-assembled using sffinfo 2.3 and newbler 2.3 (454 Life Sciences). Mate-pair sequencing and scaffolding methods are detailed in the Supplementary Methods . Interrogation of gag errors in assembled contigs Strand-specific errors similar to those recently reported [43] introduced frame-shift single-nucleotide deletion errors into ~10% of open-reading frames. These were corrected using a purpose-built algorithm, ‘bio-gag’. To investigate the properties of gag errors, Ion Torrent sequencing was carried out on isolate cultures of Bacillus amyloliquefaciens and Sulfolobus tokodaii . These data are described in a separate report [44] . De-novo assemblies using newbler 2.3 were generated and compared with their respective reference genomes (GenBank identifiers NC_014551.1 and NC_003106.2, respectively) using dnadiff (included with MUMmer, http://mummer.sourceforge.net ) version 3.22. The four bases surrounding each single-nucleotide deletion were tabulated and those contexts that contained a deletion of one base from a two-base homopolymer were considered as potential gag errors ( Supplementary Fig. 3 ). Plots were generated using Tablet [45] and ggplot2 (ref. 42) [42] . Gag errors in the Candidatus ‘ M. stordalenmirensis ’ genome were corrected with a generally applicable algorithm, presented in Supplementary Methods . Genome validation Of the 104 ortholog groups in AMPHORA2 (ref. 11) [11] , 99 were found to be single-copy groups using the ‘MarkerScanner.pl’ script of AMPHORA2 (slightly modified for implementation reasons, taking the presence of only a single peptide in the respective output fasta files to mean single copy). In addition, ndk was found using BLASTP 2.2.26+ (ref. 46 ) using the Methanocaldococcus jannaschii protein (GenBank ID NP_248261.1) as a query sequence. Two genes were interrupted by errors that appear to be gag-like. For the genes miaB and pelA , two Candidatus ‘ M. stordalenmirensis ’ peptides were reported by AMPHORA2, but in each case inspection of BLASTP against the NCBI ‘nr’ database indicated one belonged to a separate orthologous group. Thus, all 104 AMPHORA2 marker genes were found to be single copy in the Candidatus ‘ M. stordalenmirensis ’ genome. Genes thought to be single copy in Euryarchaea were also used as validation (see ‘Assessment of the Mackelprang et al. 2011 contigs’ below). Genome tree The genome tree was constructed using a concatenated protein-sequence approach using the single-copy genes in AMPHORA2 (ref. 11) [11] , with a custom Ruby script ( https://github.com/wwood/bbbin/blob/master/yagenome.rb ) git commit 3b8a124. For each of the 104 genes outlined in the Supplementary Data 1 of Wu and Scott [11] , the corresponding hidden Markov model (HMM) was queried against the protein sequences of Candidatus ‘ M. stordalenmirensis ’ using HMMER’s hmmsearch program [47] with default parameters version 3.0. The best hit protein sequence was parsed from the ‘tblout’ format using a custom biogem bio-hmmer3_report ( https://github.com/wwood/bioruby-hmmer3_report ) version 724862b and aligned to the HMM using hmmalign with parameters ‘--allcol --trim’ and the resulting stockholm format file then converted to FASTA using seqmagick git commit 6816f9d ( http://fhcrc.github.com/seqmagick ). Lowercase (unaligned) portions of the aligned sequence were then removed. These aligned sequences from each of the 104 HMMs was then concatenated into an overall Candidatus ‘ M. stordalenmirensis ’ sequence. Where no blast hit was identified, a custom biogem [41] bio-hmmer_model ( https://github.com/wwood/bioruby-hmmer_model ) version 0.0.2 was used to parse out the length of the HMM and an equivalent number of gap characters was added to the overall alignment instead. The same procedure was repeated on all finished archaeal proteomes available from IMG version 4 (ref. 36 ). A FASTA file of the overall sequences for each genome ( Supplementary Data 2 ) was used to construct a phylogenetic tree using FastTree [48] version 2.1.3 with default parameters. Sequence identifiers were then converted to a more human-readable form using the newick utils nw_rename program [49] , and visualized using Archaeopteryx [50] , ARB [51] and Inkscape ( http://inkscape.org ). Assessment of the Mackelprang et al. 2011 contigs The contig sequences for the Hess Creek genome were downloaded from NCBI (GenBank accession AGCH01000000.1). Single-copy gene analysis was carried out using AMPHORA2 (ref. 11) [11] as for the Candidatus ‘ M. stordalenmirensis ’ genome. Manual inspection of single-copy genes occurring in multiple copies confirmed the presence of multiple distinct orthologues ( Supplementary Table 7 ). Genes thought to be single copy in Euryarchaea were also used as validation, using CheckM 0.3.1 ( https://github.com/Ecogenomics/CheckM ). Out of the 136 PFAM domains found to be single copy in at least 95% of Euryarchaeal genomes, 21 were zero copy, 47 were single copy, 68 were dual copy and 1 was triple copy (estimated genome completion 85%, estimated genome contamination 50%). In contrast, the Candidatus ‘ M. stordalenmirensis ’ genome had 7 zero copy, 127 single copy and 2 dual copy (estimated genome completion 95%, estimated genome contamination 1%). To determine how many of the Hess Creek contigs were most similar to the genome of Candidatus ‘ M. stordalenmirensis ’, representative archaeal strains from IMG 4.0 ( ftp://ftp.jgi-psf.org/pub/IMG/img_core_v400/ ) [36] were chosen at random using the img_metadata_scanner.rb script of a custom-built rubygem img_scripts ( https://github.com/wwood/img_scripts version 0.0.1) with parameters ‘--sample Species Status=Finished’. This script in turn relied on another custom rubygem bio-img_metadata, version 0.0.3 ( https://github.com/wwood/bioruby-img_metadata ). The Hess Creek sequences were queried against a BLAST database made from the randomly selected concatenated genome nucleotide sequences and the Candidatus ‘ M. stordalenmirensis ’ genome using BLASTN 2.2.26+ (ref. 46 ) with default parameters. Of the 174 Hess Creek contigs, 139 showed highest similarity to the Candidatus ‘ M. stordalenmirensis ’ genome (identities 72–94%, aligned region lengths 110–10,290 bp), two were weakly (e-value >1e-6) similar to other genomes and the remaining 33 did not show similarity to any sequence in the database. On a per length basis, 31% of the Hess Creek contigs showed significant similarity to the Candidatus ‘ M. stordalenmirensis ’ genome and the reciprocal comparison showed 22% significant similarity (BLASTN e-value <1e-5, assessed using a custom script https://github.com/wwood/bbbin/blob/master/blast_overlap_percentage.rb git version 2cfaec2). The partial mcrA gene was identified in the Hess Creek contigs with TBLASTN using the Candidatus ‘ M. stordalenmirensis ’ McrA protein sequence as a query. Attempts to locate an SSU rRNA gene were performed by querying both the Candidatus ‘ M. stordalenmirensis ’ and Methanocella paludicola (IMG gene identifier 646465173) SSU rRNA gene sequences against the Hess Creek contigs using BLASTN through SequenceServer ( http://sequenceserver.com/ ). Genome annotation Genome annotation was carried out using prokka 1.5.2 (Prokka: prokaryotic genome annotation system, http://bioinformatics.net.au/software.prokka.shtml ). Genes of interest were further investigated using KEGG [52] , MetaCyc [53] , FastTree [48] , BLASTP+ (ref. 46 ) against IMG 4.0 proteomes [36] , UniRef90 (ref. 54) [54] and PFAM [55] . Metaproteomics Triplicate soil cores were collected in a sedge-dominated ( Eriophorum spp.) fen on September 1st 2010 (locations 68° 21.203 N, 19° 02.799 E; 68˚ 21.202 N, 19° 02.808 E; and 68° 21.196 N, 19° 02.808 E.). Further metaproteomic methods are detailed in the Supplementary Methods . Distribution of Candidatus ‘ M. stordalenmirensis ’ Global distribution of Candidatus ‘ M. stordalenmirensis ’ was surveyed by searching the NCBI ‘nt’ database. An overview of studies where Candidatus ‘ M. stordalenmirensis ’ was found is provided in Supplementary Tables 8 and 9 . Searching of the ‘nt’ database used BLAST 2.2.22 (ref. 56) [56] with the following parameters: ‘-v 200000 -b 200000 -p blastn -m 8’. The resultant tab-separated values file was parsed to extract hits with >97% identity using bio-table ( https://github.com/pjotrp/bioruby-table ). Hits were then downloaded from NCBI using genbank-download git version 292a2f8 ( https://bitbucket.org/simongreenhill/genbank-download/ , Greenhill unpublished) and individually used as queries to search a BLAST database consisting of the merged GreenGenes/Silva database as above, as well as the Candidatus ‘ M. stordalenmirensis ’ SSU rRNA gene region. This search was conducted using BLASTN 2.2.26+ (ref. 46 ) using the parameters ‘--max_target_seqs 1 -outfmt 6’. Those sequences that hit Candidatus ‘ M. stordalenmirensis ’ with identity >97% and could be associated with a peer-reviewed report were considered Candidatus ‘ M. stordalenmirensis ’ phylotypes. GenBank entries were linked to peer-reviewed publications using the PubMed [57] identifier present in the GenBank entry, or failing that found manually using Google Scholar ( http://scholar.google.com ) or PubMed using a combination of the ‘TITLE’ and ‘AUTHOR’ fields of the GenBank entry. Description of Candidatus ‘ M. stordalenmirensis ’ ‘ Methanoflorens ’ (Me.tha.no.flo.ren’s. N.L. n. methanum (from French n. méth ( yle ) and chemical suffix - ane ), methane; N.L. pref. methano -, pertaining to methane; N.L. masc. substantive from L. part. masc. adj. florens , flourishing, to bloom; N.L. masc. adj. ‘ Methanoflorens ’, methane producer that blooms). ‘ stordalenmirensis ’ (stor.da.len.mir.en'sis. N.L. masc. adj. ‘ stordalenmirensis ’, of or belonging to Stordalen Mire, Sweden from where the species was characterised). Methanoflorentaceae (Me.tha.no.flo.ren.ta.ce'a.e. N.L. n. ‘ Methanoflorens ’ -entis, type genus of the family; suff. -aceae, ending to denote a family; N.L. fem. pl. n. Methanoflorentaceae, the family of the genus ‘ Methanoflorens ’). Accession codes: Amplicon sequencing and metagenomic sequence data have been deposited in the sequence read archive with accession number SRA096214 . The draft ‘ M. stordalenmirensis ’ has been deposited in the integrated microbial genomes database under accession number 2518645542. Metaproteomic spectra were deposited to the ProteomeXchange Consortium ( http://proteomecentral.proteomexchange.org ) via the PRIDE partner repository under accession number PXD000410, and all metaproteomic data are published at the following URL: http://compbio.ornl.gov/stordalenmire . This website includes the metagenomic database used for MS/MS searches, p.p.m.-filtered DTASelect files and identified protein lists from each technical replicate. How to cite this article: Mondav, R. and Woodcroft, B. J. et al. Discovery of a novel methanogen prevalent in thawing permafrost. Nat. Commun. 5:3212 doi: 10.1038/ncomms4212 (2014).